Reductive assembly of cyclobutadienyl and diphosphacyclobutadienyl rings at uranium Despite the abundance of f-block–cyclopentadienyl, arene, cycloheptatrienyl and cyclo-octatetraenide complexes, cyclobutadienyl derivatives are unknown in spite of their prevalence in the d-block. Here we report that reductive [2+2]-cycloaddition reactions of diphenylacetylene and (2,2-dimethylpropylidyne)phosphine with uranium(V)-inverted sandwich 10π-toluene tetra-anion complexes results in the isolation of inverted sandwich cyclobutadienyl and diphosphacyclobutadienyl dianion uranium(IV) complexes. Computational analysis suggests that the bonding is predominantly electrostatic. Although the ψ 4 molecular orbital in the cyclobutadienyl and diphosphacyclobutadienyl ligands exhibits the correct symmetry for δ-bonding to uranium, the dominant covalent contributions arise from π-bonding involving ψ 2 and ψ 3 orbital combinations. This contrasts with uranium complexes of larger arenes and cyclo-octatetraenide, where δ-bonding dominates. This suggests that the angular requirements for uranium to bond to a small four-membered ring favours π-bonding, utilizing 5f- instead of 6d-orbitals, over δ-bonding that is favoured with larger ligands, where 6d-orbitals can become involved in the bonding. The recognition that metals can engage in π- and δ-bonding to carbocyclic ligands in addition to classical σ-bonding interactions, as exemplified by the landmark discovery of the structure of ferrocene [1] , [2] , heralded a new age of organometallic chemistry [3] . Since the inception of the field, π-ligand complexes of d-block metals with cyclo-octatetraenide, cycloheptatrienyl, arene, cyclopentadienyl and cyclobutadienyl have been investigated extensively [4] . These ligands, together with allyl and alkene ligands, constitute the important class of π-bound organometallic ligands that have proven instrumental in the development of d-orbital bonding theory. The strategy of using metals to construct and stabilize reactive π-systems has met with much success, for example, affording otherwise inaccessible organic groups, such as the square, rather than rectangular form of cyclobutadiene [5] . Furthermore, metal π-complexes find numerous applications in organic synthesis and catalysis, where complexation of a metal can increase or invert the reactivity of π-systems [6] , [7] , [8] . In the f-block, lanthanide complexes of carbocyclic π-ligands constitute a mature aspect of organolanthanide chemistry [9] , [10] , [11] . In part, this is because anionic π-ligands, such as cyclopentadienyl, bind strongly to metal centres whose bonding can be principally characterized as electrostatic. In addition, convenient synthetic methods, usually involving salt elimination, are also readily available for the straightforward installation of π-ligands, such as cyclopentadienyl and cyclo-octatetraenide, into the coordination sphere of lanthanides. For uranium, there has been intense interest in uranium π-ligand interactions because of the possibility of greater covalent metal–ligand bonding compared with the lanthanides and the implications for f-orbital bonding theory and reactivity [12] , [13] , [14] , [15] , [16] , [17] . Nonetheless, with the notable exception of cyclopentadienyl derivatives, progress has generally been hampered by a lack of synthetic methods or suitable ligand transfer reagents. The first uranium-π–ligand complex employed cyclopentadienyl in the complex [U(η 5 -C 5 H 5 ) 3 Cl], which was reported in 1956 by Wilkinson [18] , and was subsequently authenticated structurally by Yen in 1965 (ref. 19 ). This was followed by the landmark complex uranocene [U(η 8 -C 8 H 8 ) 2 ] [20] , using the cyclo-octatetraenide dianion ligand, first reported by Streitwieser in 1968 and later characterized structurally by Raymond in 1969 (ref. 21 ). The cycloheptatrienyl anions [(L) 3 U(μ-η 7 :η 7 -C 7 H 7 )U(L) 3 ] – [ L =BH 4 or NEt 2 ] and [U(η 7 -C 7 H 7 ) 2 ] – were reported by Ephritikhine [22] , [23] in 1994 and 1995, respectively, and these compounds still constitute the only examples of uranium–cycloheptatrienyl complexes in the literature. The first π-arene complex of uranium, [U(η 6 -C 6 H 6 )(AlCl 4 ) 3 ], was reported by Cesari et al . [24] in 1971, and more recently, diuranium arene inverted sandwich complexes have become prevalent [25] , [26] , [27] , [28] , [29] , [30] , [31] , [32] , [33] , [34] , [35] , [36] . However, and in contrast to the d-block, the notable exception that is absent from this series of carbocyclic π-ligands is that of cyclobutadienyl. Indeed, given the prominence of π-bound ligands in organo-f-block chemistry, it is significant and surprising to note that there are no reports of any f-block cyclobutadienyl complexes (4f or 5f). Notably, although the coupling of alkynes in the presence of uranium is well known, this typically affords acyclic chains via insertion reactions [37] , [38] , [39] , [40] . Where the reductive oligomerization of alkynes is employed, uranium-coordinated butadienyls or vinyl complexes are formed exclusively [41] . This contrasts with d-block systems that readily and efficiently execute [2+2]-cycloadditions of alkynes to give cyclobutadienyl complexes [42] . The contrasting dearth and prevalence of f-block and d-block cyclobutadienyls, respectively, suggest that orbital considerations may have an important role in overcoming the inherent strain in assembling a four-membered cyclobutadienyl ring, even when this may be offset by subsequent aromatic stabilization. However, electrostatic interactions dominate the bonding of uranium to ligand donors and, thus, steric factors may also remain important with respect to the assembly of a four-membered cyclobutadienyl ring bound to a metal centre. Herein, we show that high-valent uranium–arene complexes, supported by sterically rigid, trianionic tris( N -arylamidodimethylsilyl)methane ligands, are competent reagents for the reductive assembly of inverse sandwich uranium–cyclobutadienyl and uranium–diphosphabutadienyl complexes through formal [2+2]-cycloaddition reactions of alkyne or phospha-alkyne precursors, respectively. These complexes are the first f-block cyclobutadienyl derivatives and our studies provide insight into the chemical bonding of these systems. Synthesis Recently, as part of our work exploring triamido uranium chemistry, we reported the uranium inverse sandwich toluene complexes [{U(Ts R )} 2 (μ-η 6 :η 6 -C 6 H 5 Me)] ( 1 , R =3,5-Me 2 C 6 H 3 , Xy; 2 , R =4-MeC 6 H 4 , tol) [31] , [35] . The structural, magnetic, spectroscopic and computational data of 1 and 2 are consistent with a new class of uranium–arene complex containing uranium (V) ions and 10π-electron toluene tetra-anions. In these complexes it appears that achieving filled, closed shell ψ 4 and ψ 5 molecular orbitals of the 10π-arene, together with δ-bonding to the uranium centres, prevents oxidation of the toluene tetra-anion by uranium(V). Nevertheless, these complexes are strongly reducing, as demonstrated by the reaction of 1 with [{Co(CO) 3 (PPh 3 )} 2 ] to afford, through reductive cleavage of the cobalt-dimer and uranium(V)→uranium(IV) reduction, a uranium(IV)-cobalt bond in [U(Ts Xy )Co(CO) 3 (PPh 3 )] [31] . We thus identified these complexes as possible precursors to uranium–cyclobutadienyl complexes because of their reducing nature and the possibility of the variation of the N -aryl substituents, as the variation of ligand sterics is key to modulating f-block stability and reactivity. Addition of four equivalents of diphenylacetylene to 1 in toluene afforded a rapid colour change from red to brown. The use of fewer equivalents of diphenylacetylene resulted in very slow reactions and intractable product mixtures. When the toluene solvent is removed and replaced with hexane, and the resulting solution is stored at room temperature for 43 days, brown crystals of the diuranium–cyclobutadienyl inverse sandwich complex, a product of a formal reductive [2+2]-cycloaddition reaction, [{U(Ts Xy )} 2 (μ:η 5 η 5 -C 4 Ph 4 )] ( 3 ), are reproducibly isolated in 20% crystalline yield, Fig. 1 . Interestingly, the 1 H NMR spectrum of 3 exhibits 6 resonances for the cyclobutadienyl phenyl protons in a 4:4:4:4:2:2 ratio ( Supplementary Figure S1 ); this can be accounted for by invoking an asymmetric coordination mode of the C 4 Ph 4 2– group in solution which suggests the solid state structure ( vide infra ) is maintained in solution. Inspection of the crude toluene reaction mixture by 1 H NMR spectroscopy revealed the presence of an intermediate species ( Supplementary Figure S2 ). Despite numerous attempts, the intermediate could not be isolated, and the 1 H NMR spectrum of the crude reaction mixture cannot be assigned due to its complexity, but we suggest it is a coupled, but not ring-closed, butadienedianion similar to the bimetallic uranium–vinyl complexes recently reported by Meyer [41] . The crude mixture is formed quickly in toluene but shows only slow conversion to 3 , and it would seem that use of the less polar solvent hexane enforces precipitation of 3 , thus driving the equilibrium. The long recrystallization time may be connected with the energetic barrier associated with cyclization that must be overcome to afford 3 and may also reflect the high solubility of 3 . Notably, when the mother liquor is decanted from crystals of 3 and stored, more crystalline 3 is eventually deposited, which supports the notion that a vinyl intermediate that slowly converts to 3 is present. When 1 is treated with bis(trimethylsilyl)acetylene, no reaction is observed; although electronic considerations cannot be ignored, we suggest that the absence of reactivity with bis(trimethylsilyl)acetylene may be steric in origin. We also attempted the reaction between diphenylacetylene and 2 to give the para- tolyl analogue of 3, but this yields an intractable mixture of products that have resisted all attempts at identification. This latter observation suggests that the combination of the tetraphenyl-substituted cyclobutadienyl group with a xylyl-functionalized [U(Ts Xy )] + group represents the optimum steric combination with the tris ( N -arylamidodimethylsilyl)methane ligand set. 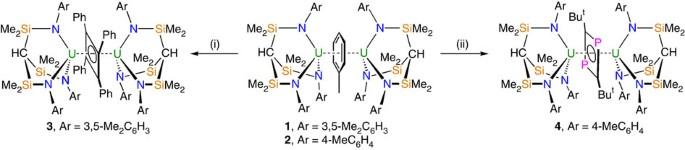Figure 1: Synthesis of 3 and 4. Reagents and conditions: (i) Toluene, 4 PhCCPh, –toluene, recrystallized from hexane, 43 days, 20%; (ii) toluene, 2 ButC≡P O(SiMe3)2, recrystallized from toluene, yield 69%. Crude1H NMR spectra obtained during the preparation and isolation of3show another species that could not be isolated, which is presumed to be a coupled butadienedianion which ring closes to give3. For the synthesis of1and2(refs31,35). Figure 1: Synthesis of 3 and 4. Reagents and conditions: (i) Toluene, 4 PhCCPh, –toluene, recrystallized from hexane, 43 days, 20%; (ii) toluene, 2 Bu t C≡P O(SiMe 3 ) 2 , recrystallized from toluene, yield 69%. Crude 1 H NMR spectra obtained during the preparation and isolation of 3 show another species that could not be isolated, which is presumed to be a coupled butadienedianion which ring closes to give 3 . For the synthesis of 1 and 2 (refs 31 , 35 ). Full size image As the reaction that afforded 3 yields the first example of an f-block cyclobutadienyl complex, but is relatively slow, we targeted a more polar triple bond in an effort to effect a more rapid [2+2]-cycloaddition reaction. We identified the phospha-alkyne Bu t C≡P as a suitable reagent due to its δ− C≡P δ+ polarization that should favour cycloaddition reactions and the isoelectronic relationship of P to a CR group. Reaction of excess Bu t C≡P with 1 does not result in the formation of [{U(Ts Xy )} 2 (μ:η 4 η 4 -C 2 P 2 Bu t 2 )]; no reaction is observed and eventually 1 decomposes on extended storage in solution; and we attribute this lack of reactivity to steric blocking as for the attempted reaction of bis(trimethylsilyl)acetylene with 1 ( vide supra ). However, replacing 1 with the sterically less demanding 2 results in a clean reaction with two equivalents of Bu t C≡P to give the diphosphacyclobutadienyl complex [{U(Ts Tol )} 2 (μ:η 4 η 4 -C 2 P 2 Bu t 2 )] ( 4 ) as red crystals in 69% yield following workup and recrystallization from toluene, Fig. 1 . The 1 H NMR spectrum for 4 is suggestive of a relatively symmetric species in solution with only six resonances observed ( Supplementary Figure S3 ), and the 31 P NMR spectrum exhibits a resonance at ~535 p.p.m. The total reaction time for the formation and isolation of 4 is ca 24 h compared with 43 days for 3 . In addition, no intermediates are observed during the formation of 4, which is in-line with the anticipated enhanced reaction rates for the polar phospha-alkyne compared with the diphenylacetylene. It would also seem that modest reduction of the steric bulk of the N -aryl groups affords sufficient space to enable tert -butyl groups to fit into the pocket between the two [U(Ts Tol )] + units, thus underscoring the importance of ligand-substituent modification for controlling the stability of the complex. Finally, the absence of any higher homologated phospha-alkyne products, for example, tri- tert -butyltriphosphabenzene, suggests that the size match of two [U(Ts Tol )] + units and (C 2 P 2 Bu t 2 ) 2– is selective for diphosphacyclobutadienyl formation. Structural characterizations The solid state structures of 3 and 4 have been determined by X-ray crystallography ( Supplementary Tables S1–S3 , and Supplementary Data 1 and 2 ) and are illustrated in Figs 2 and 3 with selected bond lengths and angles. The crystal structure of 3 reveals a dinuclear structure, where the bridging group is a tetraphenylcyclobutadienyl ligand. This is an unprecedented coordination mode for the C 4 -ring of this dianion that ordinarily binds in an η 4 -manner to one metal only [42] . Close inspection reveals that two of the phenyl rings on one side of the four-membered ring exhibit close contacts, one to each uranium (U1···C67 2.887(5), U2···C85 2.842(5) Å), to give a μ:η 5 η 5 -coordination mode overall. This enforces an asymmetric coordination of the four-membered ring that results in U–C bond distances that span a relatively wide range of 2.655(5)–2.871(5) Å. Consequently, the U–C distances between the cyclobutadienyl ring and two uranium centres fall into two pairs with bond lengths of ca 2.66 and 2.86 Å, respectively, as a result of the asymmetric coordination of the cyclobutadienyl ring, and, as a consequence, each uranium ion resides essentially midway above and below the C63–C66 bond. The U–C ipso distances (U1···C67 and U2···C85) are comparable to the longer pair of U–C ring bonds in 3 . Furthermore, although the two non-coordinated phenyl rings exhibit ispo -carbons that are in the plane of the cyclobutadienyl ring, the two ‘coordinated’ phenyl rings display C ipso carbon centres that deviate +0.61 (C67) and –0.64 (C85) Å above and below this plane. Taken together, these two features are suggestive of significant U–C ipso interactions. The cyclobutadienyl C–C distances are indistinguishable from one another and average 1.484 Å, which is fully consistent with a delocalized 6π-electron cyclobutadienyl system, as would be expected if the cyclobutadienyl ring carries a dianionic charge [43] . The U–N bond distances average 2.257 Å, which is unexceptional for uranium(IV)-amide bond lengths [44] . 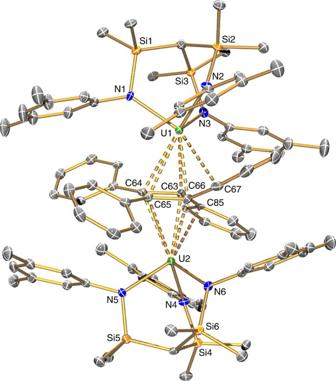Figure 2: Solid state structure of 3. Displacement ellipsoids are set to 40% probability. Lattice solvent molecules, minor disorder components and hydrogen atoms are omitted for clarity. Selected distances (Å): U1–N1 2.263(4), U1–N2 2.261(4), U1–N3 2.261(4), U2–N4 2.247(4), U2–N5 2.265(4), U2–N6 2.245(4), U1–C63 2.655(5), U1–C64 2.871(5), U1–C65 2.861(5), U1–C66 2.660(5), U1···C67 2.887(5), U2–C63 2.664(5), U2–C64 2.860(6), U2–C65 2.855(5), U2–C66 2.655(5) and U2···C85 2.842(5). Figure 2: Solid state structure of 3. Displacement ellipsoids are set to 40% probability. Lattice solvent molecules, minor disorder components and hydrogen atoms are omitted for clarity. Selected distances (Å): U1–N1 2.263(4), U1–N2 2.261(4), U1–N3 2.261(4), U2–N4 2.247(4), U2–N5 2.265(4), U2–N6 2.245(4), U1–C63 2.655(5), U1–C64 2.871(5), U1–C65 2.861(5), U1–C66 2.660(5), U1···C67 2.887(5), U2–C63 2.664(5), U2–C64 2.860(6), U2–C65 2.855(5), U2–C66 2.655(5) and U2···C85 2.842(5). 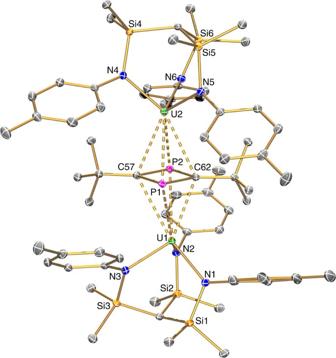Figure 3: Solid state structure of 4. Displacement ellipsoids set to 40% probability. Lattice solvent molecules, minor disorder components and hydrogen atoms are omitted for clarity. Selected distances (Å): U1–N1 2.2235(18), U1–N2 2.2337(18), U1–N3 2.2536(18), U2–N4 2.2215(18), U2–N5 2.2458(18), U2–N6 2.2241(17), U1–P1 3.0266(5), U1–P2 2.9115(5), U1–C57 2.981(2), U1–C62 2.778(2), U2–P1 3.0358(5), U2–P2 2.9081(5), U2–C57 2.866(2) and U2–C62 2.920(2). Full size image Figure 3: Solid state structure of 4. Displacement ellipsoids set to 40% probability. Lattice solvent molecules, minor disorder components and hydrogen atoms are omitted for clarity. Selected distances (Å): U1–N1 2.2235(18), U1–N2 2.2337(18), U1–N3 2.2536(18), U2–N4 2.2215(18), U2–N5 2.2458(18), U2–N6 2.2241(17), U1–P1 3.0266(5), U1–P2 2.9115(5), U1–C57 2.981(2), U1–C62 2.778(2), U2–P1 3.0358(5), U2–P2 2.9081(5), U2–C57 2.866(2) and U2–C62 2.920(2). Full size image The solid state structure of 4 is similar to 3, but clearly shows the formation of a bridging diphosphacyclobutadienyl ligand that is reminiscent of the planar [P 4 ] 2− rings found in the complexes [U(η 5 -C 5 Me 5 ){η 8 -C 8 H 6 (-1,4-SiPr i 3 ) 2 }] 2 (μ-η 2 :η 2 -P 4 ) [45] and [U{N(Ar)Bu t } 3 ] 2 (μ-η 4 :η 4 -P 4 ) (Ar=3,5-Me 2 C 6 H 3 ) [46] . The coordination mode of the four-membered P 2 C 2 ring to the uranium centres is more symmetrical than the C 4 -ring in 3 , presumably as a result of replacement of π-electron-rich phenyl rings with tert- butyl substituents. The P–C distances range from 1.794(2) to 1.810(2) Å and are indicative of a delocalized P 2 C 2 ring carrying a 2– charge. The U–P and U–C distances span the ranges 2.9081(5)–3.0358(5) Å and 2.778(2)–2.981(2) Å, respectively, and these values are in good agreement with U–P and U–C distances of ca 2.93 and 2.81 Å, typically observed in η 5 -phospholide complexes of uranium [47] . The U–N bond lengths average 2.251 Å, which compares closely to the average U–N bond length in 3 . Variable temperature magnetism In order to probe the oxidation states of the uranium ions in 3 and 4 we recorded variable temperature magnetic moment data by means of a superconducting quantum interference device (SQUID) ( Supplementary Figures S4–S7 ). The magnetic data for 3 and 4 are characteristic of uranium(IV), Fig. 4 (refs 29 , 48 , 49 , 50 ). A powdered sample of 3 exhibits a magnetic moment of 3.95 μ B at 300 K and this compares very well with a solution moment of 3.80 μ B measured in deuterated benzene solution. The magnetic moment of 3 falls to 0.67 μ B at 1.8 K. For 4 , the magnetic moment at 300 K for a powdered sample is 3.61 μ B and this decreases to 0.51 μ B at 1.8 K. The solution moment of 4 in benzene is 3.90 μ B , which is only slightly higher than the solid state moment. Both sets of magnetometric data for 3 and 4 clearly tend towards zero magnetic moments at 0 K, which suggests that both complexes contain 3 H 4 uranium(IV) centres, as tetravalent uranium has a singlet magnetic ground state. Interestingly, the magnetic moments of 3 and 4 are lower than the theoretical magnetic moment for a molecule containing two isolated uranium(IV) centres (5.06 μ B ). However, coupling of the uranium centres in 3 and 4 is not apparent from inspection of the χ versus T plots, but resolved magnetic coupling between uranium(IV) centres is very rare [49] , [50] and notoriously difficult to detect more generally for uranium, as it is usually masked by other phenomena. 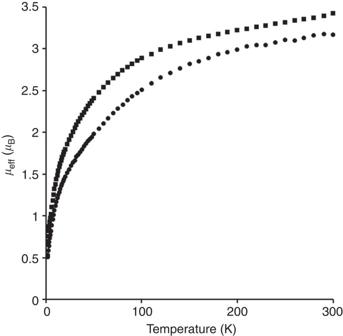Figure 4: Variable temperature magnetization data. Data for3(squares) and4(circles) recorded on a Quantum Design MPMS XL5 SQUID magnetometer. Data were recorded in an applied dc field of 0.1 T over the temperature range 1.8–300 K. Diamagnetic corrections of 1195.0 × 10−6cm3mol−1and 887.1 × 10−6cm3mol−1were applied for3and4, respectively, using tabulated Pascal constants, and measurements were corrected for the effect of the blank sample holders. Figure 4: Variable temperature magnetization data. Data for 3 (squares) and 4 (circles) recorded on a Quantum Design MPMS XL5 SQUID magnetometer. Data were recorded in an applied dc field of 0.1 T over the temperature range 1.8–300 K. Diamagnetic corrections of 1195.0 × 10 −6 cm 3 mol −1 and 887.1 × 10 −6 cm 3 mol −1 were applied for 3 and 4 , respectively, using tabulated Pascal constants, and measurements were corrected for the effect of the blank sample holders. Full size image Electronic absorption spectra We recorded the ultraviolet/visible/near infra-red electronic absorption spectra of 3 and 4 over the range 25,000–5,000 cm –1 ( Supplementary Figures S8 and S9 ). The spectra of 3 and 4 are dominated by intense absorptions in the range 25,000–10,000 cm –1 , which most likely originate from charge transfer and π–π* transitions. At lower energy, weak bands (ε<100 M –1 cm –1 ) are apparent, which can be assigned as Laporte forbidden f→f transitions. These spectra are fully consistent with the presence of uranium(IV) centres [51] in 3 and 4, which is a requirement for charge neutrality with cyclobutadienyl and diphosphacyclobutadienyl dianions. Density functional theory calculations In order to probe the electronic structures of 3 and 4 we carried out unrestricted density functional theory (DFT) calculations on the whole molecule of 3 and on a truncated model of 4 , 4a , where the diphosphacyclobutadienyl tert -butyl groups were replaced by methyl groups due to intractable convergence problems encountered with 4 ( Supplementary Tables S4–S6 ). The average calculated and experimental bond lengths for the U–C cyclobutadienyl and U–N amide interactions in 3 are in good agreement (U–C calc =2.793, U–C exp =2.760 Å and U–N calc =2.281, U–N expt =2.257 Å). For 4 , the average calculated and experimental U–N amide interactions show good agreement (U–N calc =2.253, U–N expt =2.234 Å), whereas the average calculated U–C diphosphacyclobutadienyl and U–P diphosphacyclobutadienyl distances are greater by ca 0.09 and 0.08 Å, respectively. These differences may be associated with the truncated diphosphacyclobutadienyl unit employed in the calculations for 4a . Nevertheless, given the similarity between the calculated and experimental structures for 3 and 4a, we conclude that the calculations provide qualitative descriptions of the bonding in these molecules. A comparison of calculated data for 3 and 4a is presented in Table 1 and selected α-spin Kohn Sham frontier orbitals are illustrated in Fig. 5 . Table 1 Calculated bonding and orbital parameters. 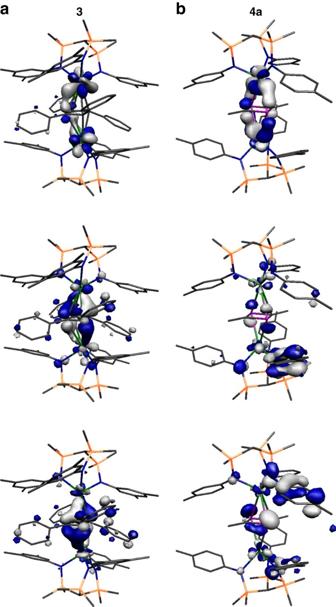Figure 5: Selected α-spin Kohn Sham frontier molecular orbitals of 3 and 4a. Top to bottom: (a) HOMO-3 (480a, −3.250 eV), HOMO-6 (477a, −4.645 eV), HOMO-7 (476a, −4.706 eV) of3; (b) HOMO-3 (392a, −3.534 eV), HOMO-6 (389a, −4.866 eV), HOMO-7 (388a, −4.941 eV) of4a. These molecular orbitals highlight the principal uranium-bridging ligand interactions in3and4a. For the compositions of these molecular orbitals, seeTable 1. Full size table Figure 5: Selected α-spin Kohn Sham frontier molecular orbitals of 3 and 4a. Top to bottom: ( a ) HOMO-3 (480a, −3.250 eV), HOMO-6 (477a, −4.645 eV), HOMO-7 (476a, −4.706 eV) of 3 ; ( b ) HOMO-3 (392a, −3.534 eV), HOMO-6 (389a, −4.866 eV), HOMO-7 (388a, −4.941 eV) of 4a . These molecular orbitals highlight the principal uranium-bridging ligand interactions in 3 and 4a . For the compositions of these molecular orbitals, see Table 1 . Full size image The calculated spin density (−2.15) and charge (+3.08) on uranium and charge on the tetraphenylcyclobutadienyl ring (−2.36) are consistent with a uranium(IV) oxidation state and tetraphenylcyclobutadienyl 2– formulation for 3 . The Nalewajski–Mrozek bond indices for the U–C cyclobutadienyl interactions (0.22–0.35, Table 1 ) and the small overlap populations between atomic orbitals on the bridging ligand and U fragments, ( Table 1 ), suggest that the bonding in 3 is dominated by electrostatic contributions with small covalent uranium–cyclobutadienyl contributions. The calculated charges for 4a (U: +3.39; dimethyldiphosphacyclobutadienyl: −2.76) and spin densities (U: −2.03) are consistent with uranium(IV) centres bound to a dimethyldiphosphacyclobutadienyl 2– ligand. Again the calculated Nalewajski–Mrozek bond orders for the U–C (0.43) and U–P (0.51) interactions, and the overlap populations ( Table 1 ), underscore the small covalent contributions to the uranium–C 2 P 2 bonding. Noting the dependency of overlap populations with the size of the basis set, we have also performed single-point calculations on 3 and 4a in which we have used a smaller basis set (double zeta basis set (DZ) from the Amsterdam Density Functional suite) for all non-U atoms. These calculations show similar magnitudes for the overlap populations ( Supplementary Table S7 ) between the U centres and the bridging ligands in 3 and 4a when compared with the calculations employing the larger double zeta, valence triple zeta, polarized basis set (TZP) basis set for all atoms ( Table 1 ). Thus, a similar description of the bonding in 3 and 4a emerges for calculations employing a smaller basis set. For 3 , the three highest occupied α-spin molecular orbitals (HOMOs) are almost entirely of uranium non-bonding 5f character. HOMO-3 (480a) reveals a modest δ-type combination between the empty ψ 4 orbital of the cyclobutadienyl ligand ( Fig. 6 ) and mainly the 5f-orbitals of the uranium centres ( Table 1 ). HOMO-6 (477a) and HOMO-7 (476a) involve uranium–cyclobutadienyl combinations that are of π-character and employ ψ 3 and ψ 2 cyclobutadienyl π-orbital combinations ( Fig. 6 ), respectively, which are usually invoked in the molecular orbital descriptions of the bonding between transition metal centres and cyclobutadienyl [5] . However, for 3, the notable difference is that the uranium 5f-orbitals are almost exclusively employed, whereas transition metals typically employ p- and d-orbital combinations. DFT calculations on 4a reveal a similar manifold as for 3 . The top three HOMOs of 4a are predominantly uranium 5f character. HOMO-3 (392a) exhibits a δ-type combination involving the empty ψ 4 orbital of the diphosphacyclobutadienyl ligand, and π-type combinations involving the ψ 2 and ψ 3 π-orbitals ( Fig. 6 ) are found for HOMO-7 (388a) and HOMO-6 (389a), respectively. 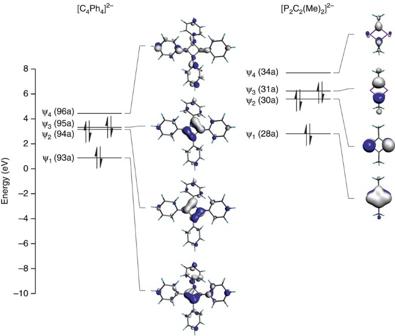Figure 6: Frontier orbitals of the cyclobutadienyl and diphosphacyclobutadienyl ligands in 3 and 4a. The ψ1-4molecular orbitals of (C4Ph4)2–and (P2C2Me2)2–were calculated by DFT at the geometries for these fragments determined by geometry optimizations for the molecules3and4a. Figure 6: Frontier orbitals of the cyclobutadienyl and diphosphacyclobutadienyl ligands in 3 and 4a. The ψ 1-4 molecular orbitals of (C 4 Ph 4 ) 2– and (P 2 C 2 Me 2 ) 2– were calculated by DFT at the geometries for these fragments determined by geometry optimizations for the molecules 3 and 4a . Full size image The orbital overlap populations ( Table 1 ) indicate that HOMO-3, HOMO-6 and HOMO-7 in 3 and 4a make little contribution to the bonding between the bridging ring and U fragments. This similarity in magnitude of the overlap populations for the δ- and π-type interactions in 3 and 4a contrasts to the situation found in uranium-inverted sandwich complexes of arenes [25] , [26] , [27] , [28] , [29] , [30] , [31] , [32] , [33] , [34] , [35] , [36] and the cyclo-octatetraenide dianion, where δ-bonding has been shown computationally to dominate for these larger aromatic systems [26] . Germane to this point, it has been noted that δ-bonding in transition metal metallocene complexes is generally weaker than in transition metal arene complexes; this is usually justified on the basis of size-matching between the metal and ligand frontier orbitals [4] . For 3 and 4a, the small overlap populations for HOMO-3, HOMO-6 and HOMO-7 may result from the relatively small size of the four-membered cyclobutadienyl and diphosphacyclobutadienyl rings, which limits the involvement of the ψ 4 , ψ 3 and ψ 2 orbitals in the bonding between these rings and uranium. The highly angular requirement of the bonding may also account for the dominance of 5f-orbital participation in the uranium-bridging ligand interactions in 3 and 4a ( Table 1 ), as well as small ligand centres such as in UE double and triple bonds (E=C, N, O) [12] , [14] , [15] , [16] , [17] , [52] , [53] , [54] . In contrast, more significant uranium 6d-orbital participation is invoked in the molecular orbital treatment of uranocene with the larger cyclo-octatetraenide ligand [55] , [56] ; here it may be that the more diffuse, less angular 6d-orbitals are better suited to bonding to spatially larger ligands. We have shown that employing highly reducing, high-valent diuranium(V) inverted arene complexes provides effective synthetic tools for preparing the first f-block cyclobutadienyl ( 3 ) and diphosphacyclobutadienyl ( 4 ) complexes. Compounds 3 and 4 are prepared by formal [2+2]-cycloaddition reactions accompanied by extrusion of toluene. For the least polar diphenylacetylene, the cycloaddition is slow, but the energetic stabilization afforded from aromaticity following cyclization eventually overcomes the inherent strain in constructing a four-membered ring, and it seems likely that two uranium centres acting cooperatively are required to effect this transformation. For the more polar phospha-alkyne, the cycloaddition is rapid. The bonding in 3 and 4 can be described as principally electrostatic, but modest δ- and π-type orbital combinations may be identified for each. The limited extent of these interactions is consistent with the relatively small size of the four-membered cyclobutadienyl and diphosphacyclobutadienyl rings. These results further our understanding of 5f-orbital bonding theory and may have applicability in designing new synthetic methodologies for the construction of novel functional group architectures. General Experiments were carried out under a dry, oxygen-free dinitrogen atmosphere using Schlenk-line and glove-box techniques. All solvents and reagents were rigorously dried and deoxygenated before use. All compounds were characterized by elemental analyses, NMR, fourier transform infra-red (FTIR) and ultraviolet/visible/near infra-red (NIR) electronic absorption spectroscopies, Evans and SQUID magnetometric methods, and single-crystal X-ray diffraction studies. Preparation of [{U(Ts Xy )} 2 (μ:η 5 η 5 -C 4 Ph 4 )] ( 3 ) Toluene (15 ml) was added to a cold (–78 °C) stirring mixture of 1 (0.83 g, 0.50 mmol) and diphenylacetylene (0.36 g, 2.00 mmol). The mixture was allowed to warm to room temperature with stirring over 16 h. All volatiles were removed in vacuo to give a brown solid. The solid was extracted into hexanes and stored at room temperature for 43 days to give crystals of 3 .0.5(PhCCPh).0.5(C 6 H 14 ) as brown blocks. Yield: 0.20 g, 20%. Anal. Cald. for C 97 H 117 N 6 Si 6 U 2 : C, 58.46; H, 6.08; N, 4.09%. Found: C, 58.48; H, 6.04; N, 3.71%. 1 H NMR (C 6 D 6 ): δ 11.81 (2H, m, p-C H -phenyl), 8.00 (4H, m, C H- phenyl), 7.63 (2H, m, C H -diphenylacetylene), 7.45 (3H, m, C H -diphenylacetylene), 6.52 (4H, br s, C H- phenyl), 6.36 (4H, br s, C H- phenyl), 4.14 (4H, s, C H- phenyl), 3.57 (2H, s, p-C H- phenyl), 1.94 (6H, br s, p-C H ), 0.13 (36H, s, C H 3 ), –0.35 (36H, s, C H 3 ), –4.21 (12H, s, o-C H ), –41.95 (2H, s, Si–C H ). Magnetic moment (Evans method, C 6 D 6 , 298 K): μ eff =3.80 μ B . FTIR v cm −1 (Nujol): 3022 (sh, s), 2280 (m), 1596 (vs), 1584 (vs), 1488 (s), 1330 (m), 1298 (br, s), 1253 (vs), 1157 (br, vs), 1094 (vbr, m), 1030 (vbr, vs), 975 (m), 888 (s), 846 (br, vs), 816 (br, vs), 754 (m), 722 (w), 700 (m), 693 (m), 672 (w), 652 (m), 565 (w), 538 (w), 497 (m). Preparation of [{U(Ts Tol )} 2 (μ:η 4 η 4 -C 2 P 2 Bu t 2 )] ( 4 ) A solution of Bu t C≡P O(SiMe 3 ) 2 (0.26 g, 1.00 mmol) in toluene (5 ml) was added slowly to a solution of 2 (0.79 g, 0.50 mmol) in toluene (10 ml) at -78 °C. The resultant mixture was allowed to warm to room temperature with stirring over 16 h. Volatiles were removed in vacuo and the solids were washed with hexanes (1 × 2 ml) then dried in vacuo to yield analytically pure 4 as a pyrophoric brown powder. Yield: 0.58 g, 69%. Red tablet-shaped crystals of 4 were grown from a saturated solution of 4 in toluene stored at –30 °C for 16 h. Anal. Cald. for C 66 H 98 N 6 P 2 Si 6 U 2 : C, 47.13; H, 5.87; N, 5.00%. Found: C, 46.86; H, 5.52; N, 4.93%. 1 H NMR (C 6 D 6 ): δ 23.37 (18H, s, Bu t ), 9.00 (12H, s, Ar–C H ), 8.81 (12H, s, Ar–C H ), 3.80 (18H, s, Ar–C H 3 ), –4.70 (36H, s, Si–C H 3 ), –69.78 (2H, s, Si–C H ). 31 P{ 1 H} NMR (C 6 D 6 ): δ 535.52 (C 2 P 2 ). Magnetic moment (Evans method, C 6 D 6 , 298 K): μ eff =3.90 μ B . FTIR v /cm −1 (Nujol): 1606 (w), 1514 (m), 1498 (vs), 1366 (s), 1300 (w), 1286 (m), 1253 (s), 1243 (s), 1211 (s), 1172 (w), 1104 (w), 1015 (br, w), 974 (m), 932 (m), 896 (m), 839 (vs), 809 (s), 764 (m), 724 (w), 710 (m), 700 (w), 544 (w), 503 (m). DFT calculations Unrestricted geometry optimizations were performed for the full model of 3 using coordinates derived from the X-ray crystal structure. Attempts to optimize the full structure of 4 resulted in intractable convergence problems in geometry optimization. Thus, we pruned the diphosphacyclobutadienyl tert- butyl groups to methyl groups in the truncated model 4a . No constraints were imposed on the structures during the geometry optimizations. The calculations were performed using the Amsterdam Density Functional suite version 2010.01 (refs 57 , 58 ). The overlap populations and orbital compositions were analysed by AOMix [59] , [60] . Further details are available in the Supplementary Methods . Accession codes: The X-ray crystallographic coordinates for structures reported in this Article have been deposited at the Cambridge Crystallographic Data Centre (CCDC), under deposition number CCDC 929447 ( 3 ) and 929448 ( 4 ). These data can be obtained free of charge from The Cambridge Crystallographic Data Centre via www.ccdc.cam.ac.uk/data_request/cif . How to cite this article: Patel, D. et al . Reductive assembly of cyclobutadienyl and diphosphacyclobutadienyl rings at uranium. Nat. Commun. 4:2323 doi: 10.1038/ncomms3323 (2013).